Historical land use change has lowered terrestrial silica mobilization Continental export of Si to the coastal zone is closely linked to the ocean carbon sink and to the dynamics of phytoplankton blooms in coastal ecosystems. Presently, however, the impact of human cultivation of the landscape on terrestrial Si fluxes remains unquantified and is not incorporated in models for terrestrial Si mobilization. In this paper, we show that land use is the most important controlling factor of Si mobilization in temperate European watersheds, with sustained cultivation (>250 years) of formerly forested areas leading to a twofold to threefold decrease in baseflow delivery of Si. This is a breakthrough in our understanding of the biogeochemical Si cycle: it shows that human cultivation of the landscape should be recognized as an important controlling factor of terrestrial Si fluxes. It has recently been shown that intense biogeochemical cycling of silica occurs in soils [1] , [2] . The annual ecosystem biogeochemical cycling of Si exceeds the annual export from continents to the ocean by two orders of magnitude [3] , [4] and effectively buffers bedrock-weathering Si fluxes [5] . Given the importance of the ecosystem biological Si buffer, human impacts on vegetation cover through land use changes will also significantly alter the biogeochemical silica cycle, although the effects on the magnitude and fluxes of silica from land to ocean are presently unknown [6] , [7] . Addressing this knowledge gap is essential, as the terrestrial silica cycle is closely connected to important terrestrial and ocean carbon sinks [8] , [9] , and to the occurrence of harmful algal blooms in adjacent coastal ecosystems [10] . Here, we show that land use is the most important controlling factor on baseflow Si mobilization in a temperate European river basin (Scheldt basin, Fig. 1 ), with historical soil disturbance and sustained cultivation (>250 years) of formerly forested areas leading to a twofold to threefold decrease in baseflow delivery of Si from the land surface to the aquatic continuum. We propose a new conceptual model in which initial deforestation leads to increased Si fluxes [11] , with sustained soil disturbance depleting soil pools of amorphous silica (ASi), eventually leading to reduced Si fluxes. These reductions add to globally important reductions in riverine Si transport by deposition in reservoirs and in eutrophicated riverine and estuarine sediments [12] , [13] , [14] . 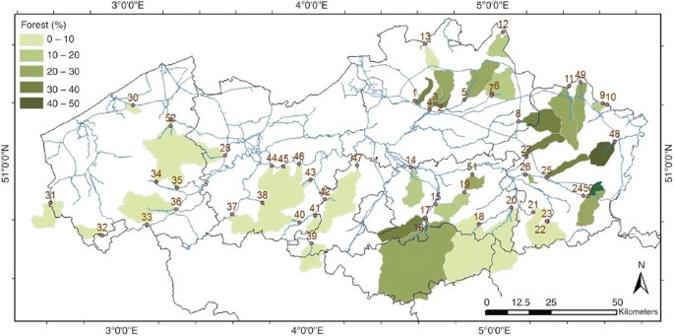Figure 1: The Belgian part of the Scheldt basin. Sampling points are indicated as red dots and numbers. Rivers draining the small watersheds are indicated in blue. The forestation degree is depicted using a green colour scale. Figure 1: The Belgian part of the Scheldt basin. Sampling points are indicated as red dots and numbers. Rivers draining the small watersheds are indicated in blue. The forestation degree is depicted using a green colour scale. Full size image Silica fluxes and concentrations Total biologically reactive silica fluxes (TSi, comprised of ASi from phytoliths and diatoms, and dissolved silicate (DSi)) were determined at baseflow in a temperate European river basin with a long agricultural history (>1,000 years; Table 1 ). The correlation between the successive TSi flux measurements (strictly speaking, log TSi flux) at the same location during our sampling campaign was 63% after correcting for land use, drainage class and soil texture effect in our linear mixed-model regression analysis. This quantitatively supports our assumption that all observations represent the long-term average baseflow conditions. Mean watershed DSi concentrations ranged from 150 to 485 μmol l −1 , whereas ASi concentrations ranged from 4 to 15 μmol l −1 ( Supplementary Data ). Si transport was completely dominated by DSi: averaged over the 51 watersheds in the Scheldt river basin, the relative contribution of ASi to TSi transport ranged from ~1.5% during summer months to ~4.5% during winter and spring months. Table 1 Characteristics of the Scheldt watershed. Full size table Effect of land use on silica fluxes Only land use ( P =0.0149) had a significant influence on the TSi fluxes. Soil texture ( P =0.3279) and drainage class ( P =0.1018) had no significant impact. 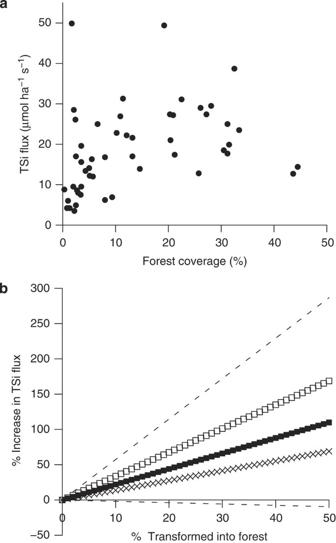Figure 2: Deforestation and Si fluxes in the Scheldt basin. (a) Variation of TSi flux (averaged per watershed, see alsoSupplementary Data) with forest cover. (b) Percentage increase in TSi flux coinciding with percentage increase in forest cover at the cost of an anthropogenic ecosystem type, as estimated from the mixed multiple linear regression analysis. The three contrasts represent the point estimates (black squares=forest versus human, open squares=forest versus grassland, crosses=forest versus cropland). The dashed upper and lower lines represent the upper (from forest versus grassland) and lower confidence intervals (from forest versus crop), respectively. The contrasts 'forest versus human' ( P =0.0214), 'forest versus agriculture (grassland+cropland)' ( P =0.0050), 'forest versus grassland' ( P =0.0023) and 'forests versus cropland' ( P <0.001) were all significantly greater than zero ( Table 2 ). The wide two-sided confidence interval for the contrast 'forest versus urban' indicates genuine uncertainty so that we cannot exclude the possibility that forests lead to a smaller TSi flux compared with urban land use. The results of Bonferroni's multiple comparison procedure to correct for multiple testing strongly support the hypothesis that forested areas have higher TSi fluxes than the other land use types ( Table 2 ). Table 2 Results of multiple regression analyses. Full size table Contrast estimates ( Table 2 ) from the regression analysis can be used to quantify the observed increase in TSi fluxes with increasing forest cover. The contrast 'forest versus human' (point estimate: 0.02173, Table 2 ) indicates that 1% of forest cover increase at the expense of a 1% decrease in human land cover results in a factorial increase of TSi flux of e 0.02173 (=1.022) or a relative increase of 2.2% of TSi fluxes. Similarly, applying all estimated significant contrasts from the analysis, the estimated relative increase in TSi flux associated with a 20% increase in forest cover is between 65% (if only grassland is replaced) and 25% (if only cropland is replaced; Fig. 2 ). The upper contrast estimates indicate an increase of more than 200% in TSi flux, with only 35% increase in forest cover. Although the lower confidence limit (as obtained from the forest versus cropland contrast) implies that we cannot fully exclude that an increase in forest coverage at the cost of cropland has no effect on TSi fluxes, the regression analysis clearly points to an overall positive effect of forests (compared with anthropogenic landscape types) on the TSi flux in the sampled rivers ( Fig. 2 ). Figure 2: Deforestation and Si fluxes in the Scheldt basin. ( a ) Variation of TSi flux (averaged per watershed, see also Supplementary Data ) with forest cover. ( b ) Percentage increase in TSi flux coinciding with percentage increase in forest cover at the cost of an anthropogenic ecosystem type, as estimated from the mixed multiple linear regression analysis. The three contrasts represent the point estimates (black squares=forest versus human, open squares=forest versus grassland, crosses=forest versus cropland). The dashed upper and lower lines represent the upper (from forest versus grassland) and lower confidence intervals (from forest versus crop), respectively. Full size image Our results differ from those of a previous study from the Hubbard Brook Experimental Forest (HBEF) [11] , in which increased export of DSi was observed up to 20 years after forest harvesting. At HBEF, increased Si fluxes were partly related to plant materials remaining on the soil surface following deforestation. In addition, mobilization and redistribution of ASi stocks occurred in the forest soils [11] . We hypothesize that the observations at HBEF and in the Scheldt basin should be interpreted as two distinct stages after the cultivation of formerly forested areas ( Fig. 3 ): HBEF is hypothesized to be representative of conditions directly after deforestation (<250 years) and the Scheldt basin is representative of sustained long-term forest soil disturbance (>250 years). 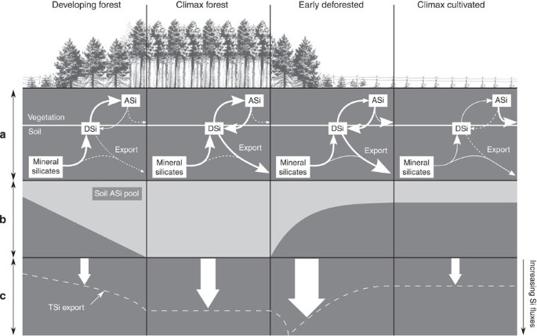Figure 3: New conceptual model for changes in Si cycling with long-term soil disturbance. (a) Hypothesized Si cycling in developing forest, climax forest, early deforested areas and equilibrium cultured areas, the associated soil ASi stock (b) and the resultant magnitude of TSi export (c). Ina, boxes represent stocks of Si. Arrows represent fluxes: the thickness of arrows is representative for flux size. Dashed arrows represent irrelevant fluxes. Inb, the light grey area represents the size of the soil ASi pool. Inc, the sizes of the arrows represent relative TSi fluxes. The dashed line represents the hypothesized evolution of the magnitude of the TSi fluxes: the closer the dashed line is to the figure bottom, the higher the TSi export (as also indicated by the arrow to the right below). ASi, amorphous Si; DSi, dissolved Si; TSi, ASi+DSi. Figure 3: New conceptual model for changes in Si cycling with long-term soil disturbance. ( a ) Hypothesized Si cycling in developing forest, climax forest, early deforested areas and equilibrium cultured areas, the associated soil ASi stock ( b ) and the resultant magnitude of TSi export ( c ). In a , boxes represent stocks of Si. Arrows represent fluxes: the thickness of arrows is representative for flux size. Dashed arrows represent irrelevant fluxes. In b , the light grey area represents the size of the soil ASi pool. In c , the sizes of the arrows represent relative TSi fluxes. The dashed line represents the hypothesized evolution of the magnitude of the TSi fluxes: the closer the dashed line is to the figure bottom, the higher the TSi export (as also indicated by the arrow to the right below). ASi, amorphous Si; DSi, dissolved Si; TSi, ASi+DSi. Full size image We therefore propose a novel conceptual model in which initial forest development is characterized by small amounts of DSi released from the soil ASi pool, compared with the amount that is annually added to the vegetation and to the soil ASi pool ( Fig. 3 ). Developing forests form net sinks for DSi: unfortunately, at present, little or no research exists that addresses Si dynamics in developing forests. An equilibrium state will eventually be reached: this stage is characterized by a large, slowly growing soil ASi stock [15] . The forest vegetation stimulates bedrock weathering of silicates through increases in soil CO 2 content, production of organic acids and stabilization of organic soil cover [16] , [17] . Trees take up the weathered DSi and deposit it as ASi plant bodies (phytoliths) in their biomass [18] . The major part of the weathered DSi passes through biomass before it is eventually released into rivers [5] . The eventual export fluxes of Si from the climax forest soils are controlled by the dissolution of soil phytoliths [19] . With deforestation, the amount of DSi exported from the forest soils drastically increases as ASi stocks dissolve [11] , [20] . However, DSi fluxes may be expected to gradually decrease again over time as there will be a fundamental imbalance: the production of biogenic ASi no longer balances the total amount of ASi dissolved, as harvesting of crops prevents replenishment of the soil ASi stock. Soil erosion will increase and ASi will be physically removed from the soils, especially during precipitation events. Increased TSi fluxes will only last until the soil reaches a new climax cultivation state, characterized by lower export TSi fluxes. The lack of deep-rooting vegetation and the absence of a significant soil organic layer restrict vegetation-stimulated weathering mechanisms. The timescale during which increases in TSi fluxes can be expected after forest cutting is currently not possible to estimate. In the HBEF [11] , increased export of DSi is still occurring 20 years after harvesting of the forest. An excess of ~16 kg DSi per year per hectare was exported from the HBEF deforested watershed, although the estimated total soil ASi pool in the integrated soil profile was about 17,000 kg ha −1 . This suggests that the increased Si flux could be sustained over ~1,000 years. The upper soil layer (O horizon) on its own contained only about 2,000 kg ha −1 , which could be depleted in about 125 years. The depletion of the ASi stocks in the lower soil horizons will likely be incomplete: several mechanisms inhibit ASi mobilization in deeper soil layers, including reprecipitation in secondary mineral silicates (for example, allophanes, immogolite, kaolinite) and incorporation of Al in phytoliths [21] , rendering them less soluble. If forest is converted to cropland, soil erosion will also remove ASi through physical erosion, thereby further reducing the timeframe during which increased DSi export can be expected. The Scheldt basin has been one of the most densely populated areas in Europe since the thirteenth century [22] . As early as 1,250, only 10% of woodland cover remained [23] ; in a pristine state, the Scheldt basin was almost fully forested (>90%). In this conceptual model, the present Scheldt basin therefore represents a new equilibrium state, which arises after forest soil ASi has been depleted or immobilized ( Fig. 3 ). Grasslands and croplands behave similarly in our data set. Grasses are known to accumulate significant amounts of ASi, resulting in the presence of a large phytolith pool in soils [1] . Yet, in our study, the grasslands were not observed to increase the downstream DSi flux. Other authors point to large phytolith stability in soils dominated by grasses [16] . This might indicate a gradual dissolution of phytoliths in forests, and a more stable phytolith pool in grasslands. Another explanation for low DSi fluxes from the Scheldt watershed grasslands is their intense management. The grasslands studied in other studies [1] consisted of natural short grass steppe and mixed and tall grass prairie communities. Such natural and seminatural grasslands cover only 0.3–0.6% of the Scheldt basin. The majority of the grassland is grazed intensively and/or mown several times a year (pastures). Furthermore, pastures are often converted into cropland within a crop rotation scheme of 3–4 years. Grazing and mowing of grasslands result in a large 'anthropogenic export' of phytoliths, and the temporary cropland stage (with increased erosion) neutralizes the positive effect of pastures on ASi accumulation. Recently established forests in Flanders often consist of conifers (pine). Acid soil conditions found in coniferous forests could increase DSi fluxes through increased weathering, but also decrease DSi fluxes from reduced ASi dissolution under acid conditions [19] . Previous studies in forested ecosystems have shown that soil ASi stocks are lower in coniferous forests compared with deciduous forests [3] . Thus, the current state of forests in Belgium is not representative of the deciduous climax forest. Another complicating factor could be the preferential reforestation on sandy soils, exhibiting higher drainage efficiency than loamy soils [24] . However, our data showed no evidence that drainage capacity had a significant impact on the observed TSi fluxes. Our results focus on baseflow mobilization of Si. Recent research in the Scheldt basin has shown that Si dynamics in agricultural watersheds change considerably during precipitation events [25] . With increasing discharge, DSi concentrations are diluted, whereas ASi concentrations rise (because of increasing transport of eroded materials). On an average, about 15–20% of total yearly transported Si from agricultural watersheds in the Scheldt basin is in the form of ASi [25] . A study in the Seine river basin also found export of ASi in soils mobilized from eroded croplands [26] . This agrees with our proposed new conceptual model, in which soil erosion increases after deforestation and ASi will be physically removed from the soils, preventing the establishment of an ASi-rich surface soil horizon. The fate of the mobilized ASi is uncertain: previous research suggests that significant amounts are deposited in wetlands [14] , [27] or lakes [12] . Preferential transport of ASi from agricultural watersheds as compared with forested watersheds might as such contribute to trapping of ASi along the aquatic continuum, an added sink for Si in continental Si cycling. The fate of ASi from harvested crops, after human sequestration, is also uncertain. Part of the ASi might be emitted again to rivers after consumption. There are, however, indications from the Seine basin that human diet constitutes only a minor part of anthropogenic point sources of Si, with most coming from detergents [26] . The fate of harvested ASi after human sequestration is a topic that should receive more attention in the future, as it might actually constitute an important part of the biogeochemical silica cycle. Despite limiting our study to baseflow conditions (60–90% of total yearly water fluxes) and the uncertainty associated with timeframes in the conceptual model ( Fig. 3 ), our data clearly indicate that long-term soil disturbance and a millennium of agricultural development have strongly changed biogeochemical Si dynamics in the Scheldt river basin (and likely in other temperate river basins). Modern agricultural practices also result in increased input of N and P to the aquatic continuum, resulting in Si limitation in aquatic ecosystems, with potentially negative effects on ecosystem quality [10] , including the development of harmful algal blooms. Our new hypothesis suggests that this DSi limitation in aquatic systems could be counteracted initially by increased Si export from cultivation of former forest soils. As the soil ASi pool gradually declines, this countereffect diminishes and Si mobilization becomes lower compared with pristine conditions. This implies that Si depletion events in more recently cultivated areas could currently still be masked by increased DSi export fluxes from recyclable ASi pools. In the Scheldt watershed, lowered Si fluxes were already attained long before intense fertilization started, and no such masking was observed. Our observations emphasize the need to increase our understanding of the effects of land use on biogeochemical Si cycling. A millennium of soil disturbance after deforestation has led to twofold to even threefold decreases in TSi flux from a watershed where the adjacent coastal zone has experienced significant eutrophication problems due to changed N:P:Si river deliveries in the last three decades [28] , [29] . Our results are the first to show that local factors controlling terrestrial Si mobilization can be separated from factors important at continental and global scales, where controlling factors largely include lithology, precipitation and slope [30] , [31] . We clearly show that land use should be included in watershed scale models for baseline Si mobilization. Our results shed new light on how historical cultivation has affected the terrestrial silica cycle, and indicate yet another anthropogenic reduction of silica fluxes through the aquatic continuum, adding to globally important reductions in riverine Si transport by deposition in reservoirs and eutrophicated rivers and estuarine sediments [12] , [13] , [14] . The observation that long-term soil disturbance has lowered baseflow mobilization of Si from landscapes is novel and part of a complex puzzle linking Si, N and P continental biogeochemical cycles to the ecological quality of coastal waters and C burial in the ocean. Transport of nutrients to the coastal zone and the ocean will be strongly dependent on processing within estuaries [32] . The yearly average filtering capacity (the ratio of the net process rate to the total inputs) of the Scheldt estuary is 0.12 for DSi, with strong seasonal fluctuations [33] . In addition, tidal marshes will have an important role in estuarine Si fluxes, especially in summer [34] , [35] . Ratios of processed nutrients in the estuary may also vary with discharge [32] . Increasing discharge lowers diatom uptake of Si within the estuary [36] , while increasing the net amount of TSi transported through the estuary [37] . Yet, the average filtering capacity demonstrates that riverine inputs of Si are an important determining factor for eventual fluxes to the coastal zone, and a good understanding of the effect of land use in Si dynamics is therefore essential. To further refine our concept of land use changes and Si dynamics, determination of germanium/silicon ratios [5] and the analysis of the isotopic Si composition [38] of river water are promising tools to trace the source of riverine DSi. These techniques may provide additional evidence for the differences in terrestrial biological control between forested and cultivated catchments. Sampling A total of 51 small watersheds (map, land use, soil texture, drainage class, river order, area, river length and average specific discharge: Supplementary Data ) were sampled in the Scheldt river basin. Lithology (quartz, feldspar) was identical for all watersheds ( Table 1 ). The selected watersheds represent all major soil series and cover the complete range of land use in the Scheldt basin. On the basis of long-term (1971–2000) observations by the Royal Meteorological Institute of Belgium (RMI/KMI), the entire study area has a temperate climate with a long-term mean annual precipitation of 820 mm and a mean January temperature of 3.1°C and a mean July temperature of 17.7°C. Major land use categories were cropland, forested land, grassland (mostly pastures) and urban land, which together cover more than 95% of land use in Flanders. Soil texture was aggregated into five classes: loam, sandy loam, light sandy loam, sand and loamy sand, and clay and heavy clay. Three drainage classes were distinguished on the basis of the depth of reduction horizons: well drained (>125 cm, class 1), moderately drained (80–125 cm, class 2) and poorly drained (<80 cm, class 3). All land use, drainage class and soil texture categories were expressed as a percentage of the total watershed area. The selected watersheds were sampled between September 2007 and October 2008 in a comprehensive, repeated (approximately every 45 days) sampling campaign of eight discrete samplings. All samples were taken near the location where the stream merges into a higher-order river and water leaves the targeted watershed. Analysis A 10 ml subsample was filtered over 0.45 μm cellulose-mixed ester filters and analysed for DSi concentration on a Thermo IRIS ICP (inductively coupled plasma spectrophotometer; Iris; detection limit 0.009 p.p.m.-Si). ASi analysis was performed on 25 ml subsamples, filtered on a 0.45 μm cellulose nitrate filter and air-dried at 20°C. Subsequently, concentrations of ASi were analysed by performing the wet chemical digestion method in 0.1 M Na 2 CO 3 on the filters [39] . Blank extractions from the filters revealed no additional Si release from the filters. Flux calculations For most of the sampling points, no discharge time series were available. Discharges were compiled from time series (1971–2008) from nearby gauging stations (<20 km) of the Flemish Environmental Agency (VMM). Topography, land use, soil texture and hydrology of these stations were similar to those of the studied watersheds. The ratio of instantaneous to long-term mean annual discharge ( Q inst / Q mean ) was assumed to follow a similar temporal pattern throughout the year at the sampling and nearby gauging location. Combining a simulated long-term mean annual discharge at the location of sampling with the known ratio of Q inst / Q mean at the nearby discharge measurement station allowed to calculate the instantaneous discharge at the sampling location at the time of sampling, as was calibrated and tested for the Scheldt basin [24] . Fluxes were then calculated by multiplying observed Si concentration with calculated instantaneous discharge. Sampling concentrated on small streams, thereby minimizing the effects of within-stream Si cycling, and was carried out during dry periods so that river discharges were near long-term average baseflow conditions (1971–2008). Our study was representative of typical baseflow conditions in the Scheldt watershed (60–90% of total yearly water flux), with negligible influence of rain-related dilution and suspended matter mobilization. The low ASi concentrations we observed during typical baseflow conditions, in all seasons, indicate that diatom uptake of DSi had negligible importance for our results. Statistics We compared forests with anthropogenic landscape elements (cropland, grassland, urban land) in a space-for-time approach, in which gradients in land use in watersheds were considered representative for the effect of long-term land use changes. We carried out a mixed multiple linear regression analysis (MIXED procedure in SAS v.9.2) with the natural logarithm of the TSi (ASi + DSi) as the response variable, and three categories of explanatory variables (land use, soil texture and drainage class). The correlation between measurements at times i and j was assumed proportional to exp(−| i − j |). Thus, we assumed an exponentially decaying correlation, with observations that are taken close to each other in time exhibiting stronger correlation than observations taken at time points that are far from each other. We also fitted a mixed multiple linear regression model assuming an autoregressive correlation pattern of order 1, which indicated virtually identical goodness-of-fit statistics and P -values as the exponentially decaying correlation. This shows that our analysis is to a large extent robust to misspecification of the correlation pattern. This regression model allows us to quantify the different effects of the four land uses (cropland, grassland, urban land and forest), while controlling for soil texture and drainage classes. It allows to test whether land use, soil texture and drainage class have a significant impact on the TSi flux, and it allows to test whether forested watersheds lead to a significantly higher TSi flux than watersheds with other land uses. To compare the impact of forests with other land uses and test our hypothesis that forested watersheds lead to higher Si fluxes than other areas, we tested the following hypotheses: Here, μ forest , μ urban , μ cropland and μ pasture represent the regression coefficients of the proportions of forested area, urban area, cropland and grasslands, respectively. We used a right-sided t -test and constructed the corresponding one-sided confidence interval for each of the contrasts μ forest − μ human (forest versus human), μ forest − μ agricultural (forest versus agriculture), μ forest − μ urban (forest versus urban), μ forest − μ grassland (forest versus grassland) and μ forest − μ cropland (forest versus cropland). The one-sided confidence interval is essentially a lower confidence limit for the value of the contrast. The degrees of freedom for the t -tests and for constructing the confidence intervals for the contrasts are determined using Satterthwaite's method. Because the one-sided confidence intervals only have a lower limit, they do not provide information regarding the largest likely values for each of the contrasts. Therefore, we also construct two-sided intervals as these do give an idea about the largest likely values for the contrasts. How to cite this article: Struyf, E. et al . Historical land use change has lowered terrestrial silica mobilization. Nat. Commun. 1:129 doi: 10.1038/ncomms1128 (2010).